Emergence of collective modes and tri-dimensional structures from epithelial confinement Many in vivo processes, including morphogenesis or tumour maturation, involve small populations of cells within a spatially restricted region. However, the basic mechanisms underlying the dynamics of confined cell assemblies remain largely to be deciphered and would greatly benefit from well-controlled in vitro experiments. Here we show that confluent epithelial cells cultured on finite population-sized domains, exhibit collective low-frequency radial displacement modes as well as stochastic global rotation reversals. A simple mathematical model, in which cells are described as persistent random walkers that adapt their motion to that of their neighbours, captures the essential characteristics of these breathing oscillations. As these epithelia mature, a tri-dimensional peripheral cell cord develops at the domain edge by differential extrusion, as a result of the additional degrees of freedom of the border cells. These results demonstrate that epithelial confinement alone can induce morphogenesis-like processes including spontaneous collective pulsations and transition from 2D to 3D. Physical confinement is well known to have a drastic influence on single-cell behaviours. For instance, constrained cancer cells in microchannels whose section is comparable to the cell size acquire a highly migrating and persistent phenotype [1] . Surprisingly, much less work has been devoted to mesoscale confinement (that is, at the scale of a small population), despite its importance in vivo . Indeed, embryonic morphogenesis proceeds mostly by rearrangements within limited cell assemblies [2] that are, for instance, related to domains of gene expression [3] . However, the collective behaviour of well-defined cell groups is also involved in other situations such as the response of cancer cell assemblies to compression [4] , [5] or the adaptation and evolution of tumours that have been proposed to be described by very generic processes [6] . On a different note, high-density new-generation cell chips operate at these mesoscales to analyse populations of a few hundred cells [7] , and tissue engineering strategies now aim at a very accurate spatial relative and absolute positioning of groups of cells of different types [8] . Experiments [9] , [10] and simulations [11] conducted on model interacting self-propelled particles have shown the importance of finite system size and the spontaneous emergence of collective behaviours. Since these types of models has successfully described the migration of cell assemblies [12] , [13] , [14] , we ask in the present article whether and how confinement alone can induce collective effects in mesoscale cell populations. By confining cells in adherent domains [15] , we show that confined epithelia exhibit collective low-frequency radial displacement modes as well as stochastic global rotation reversals. The period of these oscillations is proportional to the radius of the confining domain. A simple mathematical model, in which cells are described as persistent random walkers that adapt their motion to that of their neighbours [12] , captures the essential characteristics of these breathing oscillations. As these epithelia mature, a tri-dimensional peripheral cell cord develops at the domain edge by differential extrusion, as a result of the additional degrees of freedom of the border cells. These results demonstrate that epithelial confinement alone can induce morphogenetic-like processes including spontaneous collective pulsations and transition from two-dimensional (2D) to three-dimensional (3D) morphology. These findings are likely to have direct practical implications since the trend towards miniaturization of cell culture platforms directly results in confined small-size cell populations [7] . Confined cell monolayers Well-defined constrained monolayers with clear boundary conditions were obtained by culturing the cells on adhesive patterns within a cell-repellent surface [15] ( Fig. 1a ). We used Madin Darby Canine Kidney (MDCK) cells that develop very strong cell–cell adhesions [16] and are prototypical of epithelial cells. When these cells migrate collectively on a free surface, they spontaneously correlate their displacements over a length of typically 150 μm (roughly 10 cell sizes) [17] , [18] . Therefore, we chose to investigate domain sizes close to or smaller than this correlation length. For symmetry reasons, we used well-defined circular patterns the radii R of which varied between 50 and 200 μm. The cell-repellent surface treatment was highly effective and robust: Throughout the experiments (up to 4 weeks), cells remained on the adhesive areas and did not venture on the repellent coating ( Fig. 1a,b ). The movements of the cells were recorded within the adhesive patches, taking the confluence of the monolayer as the time origin (confluence is defined by the point at which cells have covered the entire area of the patch). 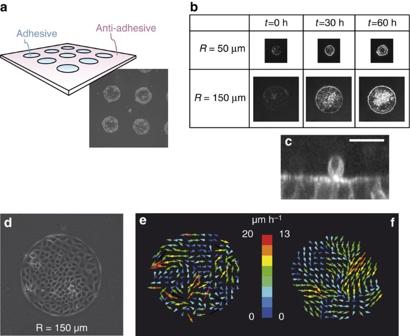Figure 1: Confined epithelium. (a) Schematics of the adhesive pattern and typical array of MDCK cell after 4 days. Cells only grow on the adhesive domains and do not venture on the non-adhesive parts of the substrate (pattern radius=125 μm). (b) Development of the monolayers with time on two different sizes of adhesive patches. The white dots in the middle of the epithelia at long times are the cells resulting from divisions that are being extruded from the monolayer when the density becomes too high. (c) Close-up on one of these extrusion events (x–z section, Lifeact cells). Scale bar, 20 μm. (d) Phase-contrast image and (e) corresponding velocity field, 6 h after confluence. (f) Simulated velocity field in the same conditions of domain size and density. Figure 1: Confined epithelium. ( a ) Schematics of the adhesive pattern and typical array of MDCK cell after 4 days. Cells only grow on the adhesive domains and do not venture on the non-adhesive parts of the substrate (pattern radius=125 μm). ( b ) Development of the monolayers with time on two different sizes of adhesive patches. The white dots in the middle of the epithelia at long times are the cells resulting from divisions that are being extruded from the monolayer when the density becomes too high. ( c ) Close-up on one of these extrusion events (x–z section, Lifeact cells). Scale bar, 20 μm. ( d ) Phase-contrast image and ( e ) corresponding velocity field, 6 h after confluence. ( f ) Simulated velocity field in the same conditions of domain size and density. Full size image The cell density increased from its nominal value at confluence (~4±2 × 10 5 cells cm − 2 ) to ~10 6 ±2 × 10 5 cells cm − 2 (s.d., n =52) in the first 30 h, as a result of cell division ( Supplementary Fig. 1A ). Cell size remained uniform across the domain during this step ( Supplementary Fig. 1B ). After 30 h, cell division slowed down but did not completely stop [19] ; the cells resulting from these divisions were apically extruded from the monolayer [20] ( Fig. 1c , Supplementary Fig. 1C,D ), a process in which cells are squeezed out of the monolayer to prevent overcrowding. Once the cells have been extruded, they remained at the surface of the monolayer without adhering to it (a gentle flow was sufficient to wash them away) and entered apoptosis [20] . Regarding cell motility, we observed the expected decrease of the average speed after confluence resulting from contact inhibition of locomotion [21] ( Fig. 2a ). Typically 30 h after confluence, the displacements within the monolayer reached a very low value ( U ≈3 μm h −1 ) and were very local [22] ( Supplementary Movies 1 and 2 ). However, compared with large monolayers studied in the same conditions, the confinement induced low-frequency velocity fluctuations that superimposed to the average decrease in speed ( Fig. 2a bars, Supplementary Fig. 2 ). The spatial distributions of the velocity modulus and the radial and orthoradial components of the velocity (respectively U r ( r , θ , t ) and U θ ( r , θ , t )) were highly non-uniform and defined homogenous areas whose size and amplitude varied wildly in space and time ( Fig. 1d,e ; Supplementary Fig. 3 ). 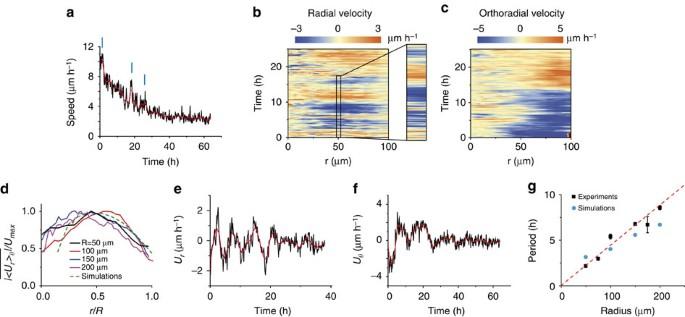Figure 2: Analysis of the velocity field. (a) Time evolution of the average speed within one representative 50 μm radius patch. Black line is the raw data. The red curve results from smoothing by adjacent averaging over 150 min. Movements become very small and local after typically 30–40 h. Note the higher velocity peaks that superimpose to the decreasing amplitude (blue bars). (b) Spatiotemporal evolution of the radial component of the velocity (averaged over all angles). Oscillations develop at mid-point between the patch centre and its edge. (c) Spatiotemporal evolution of the orthoradial component of the velocity (averaged over all angles). Cells in the domains rotate as a whole in both directions. (d) Rescaling the amplitude of the velocity radial component by its maximal value yields a universal curve against the radial coordinate normalized by the radius of the adhesive region. This curve is maximum at mid-point between the patch centre and its edge. The velocity profile resulting from simulations (average of all domain sizes) superimposes nicely with the experimental curves. (e) Oscillations ofUrwith time after angle averaging evidencing the ‘breathing’ at a period of typically 7 h (R=100 μm). The red curve results from smoothing by adjacent averaging over 100 min. (f) In contrast, fluctuations ofUθ, although of similar amplitude do not exhibit the same regularity. (g) Variations of the period of the oscillations with the size of the domain. The period was determined by Fourier transform of the time fluctuations ofUr. Error bars are the s.e. on the determination of the maximum of the peak (seeSupplementary Fig. 4A). The line is a linear fit showing the proportionality between the period of the oscillations and the radius of the patches. The blue points result from simulations performed in identical conditions. Panelsa,b,c,eandfare representative plots that were replicated 51 times over six experiments. Paneldresults from averaging 9 curves forR=50 μm, 13 curves forR=100 μm, 11 curves forR=150 μm and 2 curves forR=200 μm over a total of six experiments. Panelgresults from averaging 13 spectra forR=50 μm, 5 spectra forR=75 μm, 23 spectra forR=100 μm, 11 spectra forR=150 μm, 5 spectra forR=175 μm and 4 spectra forR=200 μm over a total of eight experiments. Figure 2: Analysis of the velocity field. ( a ) Time evolution of the average speed within one representative 50 μm radius patch. Black line is the raw data. The red curve results from smoothing by adjacent averaging over 150 min. Movements become very small and local after typically 30–40 h. Note the higher velocity peaks that superimpose to the decreasing amplitude (blue bars). ( b ) Spatiotemporal evolution of the radial component of the velocity (averaged over all angles). Oscillations develop at mid-point between the patch centre and its edge. ( c ) Spatiotemporal evolution of the orthoradial component of the velocity (averaged over all angles). Cells in the domains rotate as a whole in both directions. ( d ) Rescaling the amplitude of the velocity radial component by its maximal value yields a universal curve against the radial coordinate normalized by the radius of the adhesive region. This curve is maximum at mid-point between the patch centre and its edge. The velocity profile resulting from simulations (average of all domain sizes) superimposes nicely with the experimental curves. ( e ) Oscillations of U r with time after angle averaging evidencing the ‘breathing’ at a period of typically 7 h ( R =100 μm). The red curve results from smoothing by adjacent averaging over 100 min. ( f ) In contrast, fluctuations of U θ , although of similar amplitude do not exhibit the same regularity. ( g ) Variations of the period of the oscillations with the size of the domain. The period was determined by Fourier transform of the time fluctuations of U r . Error bars are the s.e. on the determination of the maximum of the peak (see Supplementary Fig. 4A ). The line is a linear fit showing the proportionality between the period of the oscillations and the radius of the patches. The blue points result from simulations performed in identical conditions. Panels a , b , c , e and f are representative plots that were replicated 51 times over six experiments. Panel d results from averaging 9 curves for R =50 μm, 13 curves for R =100 μm, 11 curves for R =150 μm and 2 curves for R =200 μm over a total of six experiments. Panel g results from averaging 13 spectra for R =50 μm, 5 spectra for R =75 μm, 23 spectra for R =100 μm, 11 spectra for R =150 μm, 5 spectra for R =175 μm and 4 spectra for R =200 μm over a total of eight experiments. Full size image Emergence of radial oscillations Taking advantage of the circular geometry of the adhesive domains, the two components of the velocity were angle averaged to access their mean radial spatiotemporal distributions ‹ U r › θ ( r , t ) and ‹ U θ › θ ( r , t ) ( Fig. 2b,c ). Before the epithelium entirely filled the domain, its shape was ill defined and highly fluctuating, making quantitative measurements pointless. Time averaging the absolute values of these quantities over the first 20 h after confluence showed that was minimum at r = 0 and r = R and reached its maximal intensity U r, max for r = R/ 2 ( Fig. 2d ). U r, max increased with the size of the pattern ( Supplementary Fig. 4A ). , on the other hand, was very small at the centre and maximal for r = R ( Supplementary Fig. 5A ) but did not scale with the size of the pattern, although the maximum amplitude was a decreasing function of R ( Supplementary Fig. 5B ). The dynamical variations of ‹ U r › θ and ‹ U θ › θ were obtained by averaging these quantities along r . Both components strongly fluctuated in time between positive and negative values ( Fig. 2e,f ). However, Fourier analysis showed that these fluctuations were very different in nature: no periodicity could be evidenced on ‹ U θ › θ,r ( t ); the monolayer rotated as a whole in both directions, the changes between the directions of rotation being stochastic. Of note, clockwise rotation was slightly but significantly favoured compared with counter-clockwise ( Supplementary Fig. 6 ), as already observed with other cell types [23] . This asymmetry is likely to result from intrinsic cell chirality; it is revealed here because of the relatively small and thus coherently moving cell population in presence of the adhesive/non-adhesive boundary. It is therefore a direct consequence of confinement in a domain whose size is comparable to the cell velocity–velocity correlation length [24] . In contrast, ‹ U r › θ , r clearly oscillated with time between positive (centrifugal displacements) and negative (centripetal displacements) values, at a well-defined frequency ( Fig. 2e , Supplementary Fig. 7A ), describing effectively a cooperative radial ‘breathing’ of the local displacements. The amplitudes of these displacements were typically of a few micrometres and their periods of a few hours, both quantities being a function of R ( Fig. 2g , Supplementary Fig. 4A ). Growth factors such as hepatocyte growth factor (HGF) are known to promote motility and to favour individual versus collective behaviours [25] . In the present situation, oscillations were suppressed by HGF at a concentration too low to induce scattering or enhanced proliferation in the first 12 h ( Supplementary Fig. 8D ) but sufficient to significantly affect cell–cell junctions [18] , [26] ( Supplementary Fig. 8B ). Interestingly, the average speed in the monolayer was larger in presence of this growth factor ( Supplementary Fig. 8A ). Blebbistatin also suppressed the oscillations without affecting the cell speed, emphasizing the importance of myosin II-dependent contractility in the present situation ( Supplementary Fig. 8C ). To further prove that cell division was not at the origin of these oscillations, we performed experiments in presence of mitomycin C, a drug preventing cell division. In that case, oscillations remained at the same level as in the control ( Supplementary Fig. 9A,C ). As further proof of the collective nature of these oscillations, low-calcium conditions—for which cell–cell adhesions are weakened and proliferation slowed down [27] —and HGF+mitomycin conditions were also tested. In both cases, as in the presence of HGF, the amplitude of oscillations was drastically affected ( Supplementary Fig. 9A,C ). Altogether, these results allow us to conclude that the observed oscillations are the consequence of a contractility-dependent collective effect. Oscillations have been described in different developmental and physiological processes [28] . They include the pulsed contractions of actin–myosin network [2] , [29] on time scales of the order of minutes, the ultradian oscillations with period of the order of the hour, of importance in somitogenesis [30] as well as circadian oscillations that rule the daily activity of most organisms. In the same line, propagating mitotic wavefronts resulting from mechanical signalling have been evidenced in the Drosophila embryo [31] . Since the specific mechanisms underlying these in vivo examples, and in particular the ones that involved spatial and temporal modulations of cell division, were lacking in the present study, we wondered whether breathing oscillations could be a generic outcome of collective cell motion in confined environments. Indeed, low-frequency collective modes have been reported in numerical simulations of jammed active particles in confined domains with a period set by the system size [11] . Here, however, in contrast with these previous simulations, the oscillations took place before the monolayer reached the jammed, glassy state identified in refs 32 , 33 . Cells were still very mobile, did not rotate in a ‘cage’ made by their neighbours and did not exhibit anomalous density fluctuations ( Supplementary Fig. 10 ). The present oscillations appeared also quite distinct from the mechanically excited waves in large size, unconfined, migrating epitheliums reported in ref. 27 . Indeed, in this last case, the migration-induced mechanical waves propagated roughly parallel to the local cell motion and two waves appeared to traverse each other like solitary waves. On the contrary, the present oscillation modes were observed for the radial velocity, whereas, because of confinement, the cells moved preferentially in the orthoradial direction. The oscillation patterns appeared horizontal in the spatiotemporal plots ( Fig. 2b ), indicating a global oscillation. We estimated this effect by measuring a difference of phase between different radial positions from these heatmaps (see Methods). We found that this dephasing was not significantly different from zero ( t -test, n =50), confirming the global character of these oscillations. A particle-based model describes well the radial oscillations In a previous study [12] , we have shown that collective migration of the same MDCK cells that were used in the present study, was well described by a simple mathematical model in which cells were described as persistent random walkers having a tendency to adapt their velocities to that of their neighbours. In addition, each cell was repelled at short distance by its neighbours to prevent cell overlap, and felt some attraction towards them in an intermediate range of distance to crudely mimic cell adhesion and epithelium cohesiveness. This approach was originally proposed by Vicsek et al. [34] as a characteristic property of collective motion in general and was incorporated since then in various models of collective cell motion [12] , [13] , [35] . Therefore, we found it interesting to investigate whether low-frequency breathing oscillations would be present in simulations of the model of ref. 12 in a confined domain. Since cell division was shown to be dispensable in the experiments, it was not implemented in the simulations and cell density was fixed at 6 × 10 5 cells cm −2 comparable to that of the experiments during the breathing oscillations (see Methods section for a detailed description of the model and simulations). As shown in Fig. 1e,f , the simulated velocity fields visually resembled the experimentally observed ones, as already observed in ref. 12 , although cell speeds were slightly smaller. The spatiotemporal variations of the radial and orthoradial components of the velocity were very close to the experimental ones ( Supplementary Fig. 11 versus Fig. 2b–d ; Supplementary Fig. 5A versus Supplementary Fig. 5C ; Fig. 2d ). In particular, very similar breathing oscillations were observed in the simulations ( Supplementary Fig. 4B ) and in the experiments ( Fig. 2e ). In both cases, the period increased linearly with the domain size. Moreover, the simulated and experimentally observed frequencies in different domain sizes quantitatively agreed ( Fig. 2g ). We therefore conclude that the observed breathing oscillations do not require a specific mechanism to emerge, in contrast, for instance, with the models of mechanically excitable waves proposed in ref. 27 or ref. 31 , but are the natural consequence of oscillatory modes in a confined domain excited by the spontaneous stochastic motions of the cells. This result highlights that the pattern-induced finite size effect is sufficient to trigger size-dependent oscillations. Therefore, we believe that confining the cells in the patterns fixes the size of the epithelium but does not play an ‘active’ role, for example, by inducing a specific signal for the oscillations of the epithelium. Similarly, the global orthoradial displacements and the stochastic reversals in the orthoradial velocity U θ ( Supplementary Figs 6B and 12 ) appear as generic consequences of velocity alignment and stochasticity on the unhindered global rotation mode. Formation of a tri-dimensional peripheral rim We now turn to the later stages of these highly confined monolayers ( t >25 h). When the density reached a value of ~10 6 cells cm − 2 , the increase in population within the monolayer drastically slowed down [19] ( Supplementary Fig. 1C,D ). In the centre of the domains, the divisions still occurring resulted in the extrusion of the newly generated cells out of the monolayer where they remained without adhering to it [20] ( Fig. 1c ). These cells were readily rinsed by a modest flow such as the one used for renewing the medium. Except for this contribution, the system remained bi-dimensional. However, next to the border of the adhesive patch, the tissue systematically formed a tri-dimensional peripheral cell cord (a ‘rim’) all along this edge ( Fig. 3a,b ) that can be identified in phase-contrast images by a white ring corresponding to its inside edge ( Supplementary Fig. 13A ; observation repeated on 100 domains from six independent experiments). Rims grew at a rate compatible with the cell division rate at the onset of rim formation ( Fig. 3d,e ). To test whether a centrifugal cell flow could be involved in the formation of these rims, we measured the radial cell flow from the radial velocity near the edge at the onset of their appearance. We found that the contribution to the growth of the rim originating from a centrifugal flow was at least 10 times smaller than its actual growth rate ( Supplementary Fig. 14 ; 0.2±0.1 μm h −1 (s.d. ), n =42, over four experiments). Therefore, these rims resulted mostly from proliferation, not from centrifugal net cell flow. 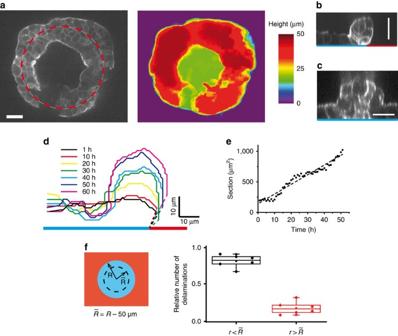Figure 3: Development of a tri-dimensional peripheral rim. (a) Confocal section 15 μm above the basal plane showing axysection of the rim (left panel). Actin-green fluorescent protein cells. The dashed line is the limit of the adhesive patch in thez=0 plane. The right panel is a colour-coded 3D reconstruction of the same domain. Scale bar, 20 μm. (b)xzsection of the rim. The blue line figures the adhesive treatment and the red one, the non-adhesive treatment (R=50 μm,t=72 h). Note the cell overhang over the non-adhesive substrate; 50 replicates. Scale bar, 20 μm. (c) ‘Bulge’ developing on top of the monolayer. Its structure and size are close to the outer rim (t=72 h) Scale bar, 20 μm. (d,e) Dynamics of development of the rim. (R=50 μm). Representative plots, two replicates. (f) Relative number of extrusions in the centre versus the border, showing that individual delaminations are mostly located in the centre. Results of divisions at the periphery are incorporated in the rim. (P<10−6, two-samplet-test).R=100 μm andR=200 μm.n=50 over five experiments. Box limits are first and third quartiles, inside line is the median. Whiskers lengths are the outermost data point that falls within 1.5 interquartile range of the lower quartile, and within 1.5 interquartile range of the upper quartile. Figure 3: Development of a tri-dimensional peripheral rim. ( a ) Confocal section 15 μm above the basal plane showing a xy section of the rim (left panel). Actin-green fluorescent protein cells. The dashed line is the limit of the adhesive patch in the z =0 plane. The right panel is a colour-coded 3D reconstruction of the same domain. Scale bar, 20 μm. ( b ) xz section of the rim. The blue line figures the adhesive treatment and the red one, the non-adhesive treatment ( R =50 μm, t =72 h). Note the cell overhang over the non-adhesive substrate; 50 replicates. Scale bar, 20 μm. ( c ) ‘Bulge’ developing on top of the monolayer. Its structure and size are close to the outer rim ( t =72 h) Scale bar, 20 μm. ( d , e ) Dynamics of development of the rim. ( R =50 μm). Representative plots, two replicates. ( f ) Relative number of extrusions in the centre versus the border , showing that individual delaminations are mostly located in the centre. Results of divisions at the periphery are incorporated in the rim. ( P <10 −6 , two-sample t -test). R =100 μm and R =200 μm. n =50 over five experiments. Box limits are first and third quartiles, inside line is the median. Whiskers lengths are the outermost data point that falls within 1.5 interquartile range of the lower quartile, and within 1.5 interquartile range of the upper quartile. Full size image During these experiments, it was very clear that individual extrusions resulting in loss of cells occurred almost exclusively at the centre of the domains and not at the area occupied by the rim. This is directly visible for instance in Fig. 1b at long times where the extruded cells that appear as white dots on the images are much more numerous in the centre of the domains than at their periphery. This observation was quantified by counting these individual extrusion events in the central and peripheral areas. Rates of extrusion in the peripheral region were found to be more than four times smaller than in the central region ( Fig. 3f ). We call this phenomenon ‘differential extrusion’. Edge enhancement of proliferation has been reported for endothelial cells in confined geometries after several days [36] . Although in the present experiments, there was no evidence of such a phenomenon in the first 25 h after confluence ( Supplementary Fig. 15 ), we do not exclude a similar effect at longer times. However, we emphasize the importance of differential extrusion by which divisions occurring in the rim contribute to its growth, whereas divisions in the centre are individually extruded before entering apoptosis. Rims were systematically observed on domains of all sizes. Their widths did not depend on the domain size ( Supplementary Fig. 13A ) and they merged into a single circular aggregate (a ‘droplet’) for radii smaller than the typical rim width (~20 μm; Supplementary Fig. 13B,C ). The development of these 3D structures from monolayers of MDCK cells that are commonly viewed as the prototype of the bi-dimensional epithelial phenotype is another surprising outcome of the confinement. It is an intrinsic response of the epithelium to a boundary regardless of its exact geometry. Apico-basal polarity was probed with ezrin as an apical marker. It developed in the monolayer as soon as confluence was reached. At the rim, the polarity developed similarly at a multicellular scale with a well-defined apical side at the rim–solution interface ( Fig. 4 ). The apico-basal polarization was systematically larger at the rim than in the monolayer ( Fig. 4c,d , Supplementary Fig. 16 ). These peripheral cords polarized globally and behaved in this respect as single coherent pluricellular structures. In particular, some cells belonging to the rim showed a clear ezrin-rich apical side, although they did not directly interact with the substrate ( Fig. 4d ). Also, cells belonging to the rim remained alive as long as culture conditions were maintained, in contrast with the individually extruded cells that quickly enter apoptosis [20] . Therefore, we show here that concerted cell–cell contacts can compensate for lack of engagement of the cells with the underlying substrate that causes cell death [20] . 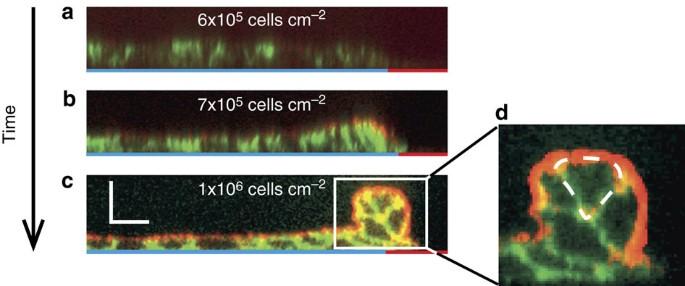Figure 4: Establishment of apico-basal polarity. Ezrin (red) is an apical marker. E-cadherins (green) label the cell–cell junctions. (a–c) As density increases, the monolayer polarizes. As can be assessed fromc, at high densities, the rim is more polarized than the monolayer (Supplementary Fig. 16). Scale bars, 10 μm. (d) Close-up ofcwith a different balance of colours. The polarity of the rim is global (that is, at the scale of the structure), allowing defining a ‘collective polarity’ (seeSupplementary Fig. 16). Note that some cells are polarized, although they do not interact with the substrate but only with other cells (dash line). Representative image, 20 replicates in two experiments. Figure 4: Establishment of apico-basal polarity. Ezrin (red) is an apical marker. E-cadherins (green) label the cell–cell junctions. ( a – c ) As density increases, the monolayer polarizes. As can be assessed from c , at high densities, the rim is more polarized than the monolayer ( Supplementary Fig. 16 ). Scale bars, 10 μm. ( d ) Close-up of c with a different balance of colours. The polarity of the rim is global (that is, at the scale of the structure), allowing defining a ‘collective polarity’ (see Supplementary Fig. 16 ). Note that some cells are polarized, although they do not interact with the substrate but only with other cells (dash line). Representative image, 20 replicates in two experiments. Full size image We propose that differential extrusion and, as a consequence rim formation, results from an unbalance of the mechanical forces acting on the border cells as they divide in the mechanically constrained environment of a dense monolayer: at the early stages, cells resulting from divisions are incorporated in the monolayer as cell density increases ( Fig. 5a ), but above typically 10 6 cells cm − 2 , the monolayer can no longer compress and these cells are apically extruded [20] ( Figs 1b,c and 5b ; Supplementary Movie 3 ). At the edge of the domains, however, the cells are constrained by the repellent coating only at their ventral side; their lateral side facing the cell-free surface keeps some flexibility and can deform in response to division ( Fig. 5c ; Supplementary Movie 4 ). Of note, structures similar to the rim occasionally appeared at the surface of the monolayer ( Fig. 3c ) for patches larger than 100 μm. These ‘bulges’ developed simultaneously as the rims in ~50% of the patches (25 observations from 43 domains in six independent experiments). They resulted from divisions that have managed to exploit the remaining limited flexibility still present at these high densities. 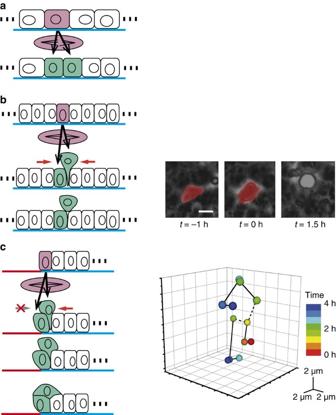Figure 5: Mechanism of rim formation. (a) At relatively low densities, the division of a cell in the monolayer results in an increase of the density. (b) Above a certain density threshold, density cannot increase anymore and results of cell division are extruded from the monolayer. Eventually, these cells enter apoptosis. On the image’s sequence,t=0 corresponds to mitosis. Scale bar, 10 μm. (c) At the domain border, cells incorporate better in the rim. The additional degrees of freedom allow a tri-dimensional rim to develop. The 3D plot is a trajectory of the nuclei (H2B-mCherry cell line) of a mother and its two daughter cells. After division, one of the daughters goes to the basal plane while the other moves to the upper part of the rim. Representative plot, 30 replicates in two experiments. See alsoSupplementary Movies 3 and 4. Figure 5: Mechanism of rim formation. ( a ) At relatively low densities, the division of a cell in the monolayer results in an increase of the density. ( b ) Above a certain density threshold, density cannot increase anymore and results of cell division are extruded from the monolayer. Eventually, these cells enter apoptosis. On the image’s sequence, t =0 corresponds to mitosis. Scale bar, 10 μm. ( c ) At the domain border, cells incorporate better in the rim. The additional degrees of freedom allow a tri-dimensional rim to develop. The 3D plot is a trajectory of the nuclei (H2B-mCherry cell line) of a mother and its two daughter cells. After division, one of the daughters goes to the basal plane while the other moves to the upper part of the rim. Representative plot, 30 replicates in two experiments. See also Supplementary Movies 3 and 4 . Full size image As could be expected for such collective phenomena, HGF suppressed these 3D structures (bulges and rims): they did form initially similar to the control experiments but quickly destabilized as more cells got extruded from the monolayer ( Supplementary Fig. 17 ), presumably as a result of large cell densities (80 h after HGF treatment, no rim was observed on any of the 30 analysed domains). Blebbistatin in contrast destabilized only the monolayer bulges but not the peripheral cell cords ( n =18 domains; Supplementary Fig. 18A ). Moreover, myosin inhibition did not impair rim formation when the drug was added 14 h after confluence (~10 h before expected rim formation). Rims then formed and developed similarly as in the absence of inhibition ( n =18 domains; Supplementary Fig. 18B ). This result demonstrates the stabilizing role of the edges even in the absence of contractility. Formation of cell cords is routinely observed with cells derived from blood vessels or kidney—as are the MDCK studied here—in 3D environments, in presence of growth factors [37] . 2D confinement at the cell scale has been previously evidenced to favour the formation of cysts in Matrigel [38] . Cord formation has also been observed for human umbilical vein endothelial cells on adherent stripes of width smaller than 50 μm in the absence of gel or other 3D environment [39] . Our own work confirms that geometrical cues are sufficient to trigger morphogenetic mechanisms at the very early stages of the formation of the organ itself. Note however that, here, the polarity is inverted compared with the gel situation, a situation often encountered with MDCK cells cultured in suspension [40] . Moreover, a single well-defined boundary is enough to define the cell cord, the dense monolayer itself participating actively to the formation and stabilization of this structure. Several models based on non-uniform cell growth across growing islets have emphasized the role of free edges [41] , [42] , [43] , [44] , [45] , some of them resulting in out-of-plane modulations [41] . Our results do not exclude these mechanisms by which more cells get to be produced at peripheral regions. However, we show here that differential extrusion appears to be a crucial mechanism by which new cells resulting from divisions get to be incorporated preferentially at the periphery of constrained tissues, favouring this way the development of 3D structures or cords. It is commonly believed that gels or 3D environments are necessary to the formation of cell cords. The present results widen this view by showing that gels are not necessary to initiate cord formation (although they may accelerate this process). Further, relatively large-scale confinement is efficient in the development of these structures via (i) the presence of well-defined borders and (ii) high cell densities. Cell cords are therefore the consequence of interacting cells in presence of a physical boundary. Obviously, 3D environments become extremely important in the following stages of lumen formation [37] , [46] . Finally, we note that well-defined adhesive domains of small sizes are basic constitutive elements of new-generation cell chips. We have demonstrated here that such domains may promote unusual collective cell dynamics and the spontaneous emergence of structures at the domain rim. We expect that both will have to be taken into account in the future developments of lab-on-chip techniques. Preparation of the patterns Glass slides were first PEGylated with a particularly robust surface treatment [15] . Domains were defined by photolithography directly on the cell-repellent coating in such a way that it remained protected by the photoresist everywhere except at the desired location of the adhesive domains. Using the photoresist as a mask, the polyethylene glycol (PEG) coating was etched on the photoresist-free areas with an air plasma, revealing the underlying glass. The resist was then dissolved away leading to clean glass domains surrounded by PEG-coated glass. Cell culture MDCK cells [47] were cultured in DMEM supplemented with 10% fetal bovine serum (Sigma), 2 mM L -glutamin solution (Gibco) and 1% antibiotic solution (penicillin (10,000 units ml −1 ), streptomycin (10 mg ml −1 )). Cells were seeded and maintained at 37 °C, 5% CO 2 and 90% humidity throughout the experiments. We also used actin-green fluorescent protein cells [48] and Lifeact cells (prepared by O Cochet-Escartin) [49] for imaging actin as well as clones expressing histones H2B-mCherry [50] for the density measurements (these clones were cultured in presence of geneticin (400 μg ml −1 )). Typically, 10–100 cells were initially seeded in each pattern. The exact number of cells initially plated did not influence the end result ( Supplementary Fig. 19 ). Unless otherwise specified, drugs were added 12 h post confluence. In mitomycin inhibition experiments, Hoechst NucBlue Live ReadyProbes Reagent (Life Technologies) was added 11 h after inhibition to label nuclei. HGF (Sigma), mitomycin c (Sigma) and Blebbistatin (Sigma) were used respectively at a concentration of 10 ng ml −1 , 5 μg ml −1 and 50 μM. In that case, experiments were started in the absence of drug. A fraction of the supernatant was pumped out at the chosen time, mixed with the drug and re-injected in the well. When using mitomycin, signs of toxicity were observed 12–13 h after adding the drug and the experiment was stopped at that point. We also used a low-calcium medium to reduce cell–cell adhesions (calcium-free DMEM, fetal bovine serum 10%, Penstrep 1%, 50 μM calcium). We first cultured the cells in regular DMEM and changed the buffer to low-calcium DMEM 12 h after the confluence. Microscopy and data analysis Patterned glass slides were glued at the bottom of a pre-drilled Petri dish or a six-well plate, using a silicone elastomer (Sylgard 184; Dow Corning), and then cured 5 min at 90 °C on a hot plate. Starting from seeding, the cells were imaged in phase contrast on an Olympus IX71 inverted microscope equipped with a temperature, CO 2 and humidity regulation (LIS), a motorized stage for multipositioning (Prior) and a CoolSNAP HQ2 camera (Roper Scientific). Unless otherwise specified, a × 20 objective was used and images were acquired every 10 min. Displacements and image acquisition were computer controlled with Metamorph (Molecular Devices). The 3D structures that eventually developed in the monolayer were observed with the actin-green fluorescent protein cells, the Lifeact cells or the H2B-mCherry cells in confocal microscopy using an Eclipse Ti microscope (Nikon) equipped with a Roper spinning disk. Hoechst-labelled cells were observed in wide-field fluorescence microscopy (Olympus IX71). Cadherin and ezrin were imaged on fixed cells by immunofluorescence: for cadherins, cells were labelled with a mouse anti-Ecadh (BD, 1/400) coupled to a goat anti-mouse Alexa Fluor 488 (Life Technologies, 1/1,000); for ezrin, cells were labelled with a rabbit anti-ezrin (from Monique Arpin, UMR144, Institut Curie, Paris, France), (1/600) and then coupled to a goat anti-rabbit Alexa Fluor 568 (Life Technologies, 1/500). Observations were performed in confocal microscopy. The apico-basal polarity was determined from the localization of ezrin. We measured the basal and apical levels of fluorescence (respectively α b and α a —these quantity were background corrected) and defined the contrast as . Image processing was performed with custom Matlab (Mathworks) routines. In particular, the velocity field was mapped by particle image velocimetry [22] . PIV parameters were chosen as follows: subwindows size=12 μm; overlap=75%. We checked that our results were robust regarding these parameters and consistent with manual tracking on several examples. Subsequent data analysis was performed with Matlab or Origin (Originlab). Density fluctuations were computed using Matlab by measuring the number of cells in subwindows of increasing sizes. From these measurements, we extract the average value and the s.d. In Supplementary Movie 4 , the height of the nuclei is colour coded and the different levels are visible on the same image. Differences of phase in the oscillations at different locations along the radius were measured from the radial velocity heatmaps. They were first smoothed, thresholded and filtered, and then the orientation of each domain with the horizontal was assessed by the ‘regionprops’ Matlab routine. Simulations The simulated model is based on the model developed in ref. 12 and described in detail below. In our previous work [12] , we wished to try and accurately describe the motion of MDCK cells in an actively moving epithelium with as simple a model as possible. The description of each cell was reduced to its centre point and assumed to be a persistent random walk biased by its interaction with the immediately neighbouring cells. We found it possible to quantitatively reproduce the cell motions in our experiments by suitably adjusting the parameters of this simple model. In the present work, we have thus implemented this previously proposed model with the parameters determined in ref. 12 . A repulsive boundary force has simply been added to mimic the cell-repellent surface. The model is formulated as follows. An epithelium consisting of N cells is described by a collection of N point particles (that is, the N cell centres). Each particle has a position r i and moves with a velocity v i , where the particle index i runs from 1 to N. The velocity v i of the cell i is a real 2D vector that evolves as: The meaning of the different terms on the right-hand side of equation (1) is as follows. The linear damping term (− α v i ) accounts in an effective way for the fact that cell motion is a dissipative process and effectively endows the velocity dynamics with an exponential memory kernel on a time scale 1/ α . The motion of cell i is influenced by its interaction with its neighbours as reflected by the summation sign on the right-hand side of equation (1). The sum is performed on the N i cells j that are the nearest neighbours of cell i , namely, the cells that are supposed to be in direct contact with cell i . This interaction between a cell and its neighbours takes place in two ways. First, the velocity of cell i tends to become equal to the velocity of the neighbouring cell j with a strength determined by the coupling constant β as proposed as a general feature of collective motion in ref. 34 . Second, the fact that cells do not overlap and adhere to their neighbours is taken into account by the force f ij between neighbouring cells i and j . The force f ij is repulsive with a hard core at short distances and attractive at longer distances up to maximal distance a m at which cells cease to interact even if they are topological nearest neighbours. It is taken under the form with r ij =| r i − r j |. The potential U(r) is chosen as the sum of a repulsive short-range Gaussian potential and an attractive part acting at longer distances: with, as in ref. 12 U 0 =2,400 μm 2 h −2 , a 0 =8 μm , U 1 =2 h −2 , a 1 =35 μm , a m =80 μm and H(x) the Heaviside function, H(x) =1 for x >0 and H(x) =0 otherwise. Neighbours of a cell/particle need to be defined to implement equation (1). For computational simplicity, this is done as follows. The neighbourhood of a particle i is split into six equal sectors (with the x axis taken as one of the sector boundaries). The particle closest to particle i in each sector is taken to be a neighbour of particle i if its distance to particle i is less than a m =80 μm. The stochastic motion of each cell arises from the noise term η i in equation (1). It is taken to be an Ornstein–Uhlenbeck process with correlation time τ: with ξ i a delta-correlated white noise independently drawn in each cell , where α and β stand for the ( x , y ) coordinate indices. Finally, the external repellent surface is a specific feature of the present work. It is described by the external repulsive f ext in equation (1), which is taken as with a e =4 μm and r e related to the radius of the adhesive disk in the modelled experiment, as explained below. All the results reported in the main manuscript were performed with the parameters determined in ref. 12 , that is, Cell division was not implemented in the model. The simulations were performed at a fixed density of 6 10 5 cells cm − 2 , representative of the cell density during the breathing mode period. To model a disk of radius R , the external radius r e was chosen so that the (fictitious) edge of the external cells would be at R . The four different simulation sizes reported in the main manuscript were thus performed with ( R, r e , N )=(50 μm, 46.4 μm, 47); (100 μm, 96.3 μm, 188); (150 μm, 146.4 μm, 424) and (200 μm, 196.5 μm, 754). Some supplementary simulations were performed to quantify the influence of the velocity alignment term on the cell population mean radial velocity dynamics ( Supplementary Fig. 9B ). In this case, equation (1) was replaced by Note that the direct influence of the neighbouring cell velocities on a cell own velocity was eliminated, but that the damping effect of the β term was kept so that cells had comparable velocities with or without alignment interaction. All the other parameters were kept unchanged. The three sets of simulations of Supplementary Fig. 9B were performed as those of the main text with ( R, r e , N )=(100 μm, 96.3 μm, 188); (150 μm, 146.4 μm, 424) and (200 μm, 196.5 μm, 754). How to cite this article: Deforet, M. et al. Emergence of collective modes and tri-dimensional structures from epithelial confinement. Nat. Commun. 5:3747 doi: 10.1038/ncomms4747 (2014).